Redox active iron nitrosyl units in proton reduction electrocatalysis Base metal, molecular catalysts for the fundamental process of conversion of protons and electrons to dihydrogen, remain a substantial synthetic goal related to a sustainable energy future. Here we report a diiron complex with bridging thiolates in the butterfly shape of the 2Fe2S core of the [FeFe]-hydrogenase active site but with nitrosyl rather than carbonyl or cyanide ligands. This binuclear [(NO)Fe(N 2 S 2 )Fe(NO) 2 ] + complex maintains structural integrity in two redox levels; it consists of a (N 2 S 2 )Fe(NO) complex (N 2 S 2 =N,N′-bis(2-mercaptoethyl)-1,4-diazacycloheptane) that serves as redox active metallodithiolato bidentate ligand to a redox active dinitrosyl iron unit, Fe(NO) 2 . Experimental and theoretical methods demonstrate the accommodation of redox levels in both components of the complex, each involving electronically versatile nitrosyl ligands. An interplay of orbital mixing between the Fe(NO) and Fe(NO) 2 sites and within the iron nitrosyl bonds in each moiety is revealed, accounting for the interactions that facilitate electron uptake, storage and proton reduction. Hundreds of diiron carbonyl complexes of the forms (μ-SRS)[Fe I (CO) 3 ] 2 and (μ-SRS)[Fe I (CO) 2 L] 2 have been synthesized in recent years as synthetic analogues of the 2Fe subsite within the 6Fe cluster that is the active site of the remarkable hydrogen-producing biocatalyst, [FeFe]-hydrogenase, [FeFe]-H 2 ase (ref. 1 ) ( Fig. 1 ). Many have been established as modest solution electrocatalysts for H 2 production, while others have served to benchmark spectroscopic signatures related to redox levels within the natural enzyme [2] , [3] , [4] , [5] , [6] . In addition to the diatomic CO and CN − ligands, the features of the [FeFe]-H 2 ase active site that are replicated throughout these models are typically the bridging dithiolate, which aids in maintaining the butterfly shape of the 2Fe2S core and the close proximity of the two irons, within a metal–metal bonding distance of ca. 2.5 Å. In this way, two base metals in a single unit can share the required redox changes and perform two-electron catalytic functions as do single noble metals such as Pt 0 or Pd 0 , currently used in hydrogen technology. The search for mechanistic understanding of the electrocatalysis by the active site models has inspired informative computational studies [7] that intimate the roles of each component of the deceptively simple active site. Biochemical studies have shown that the redox active 4Fe4S cluster that is directly attached to the 2Fe subsite is required for the extraordinary activity of the enzyme. However, intricate molecular constructions with exogeneous redox active centres attached to the diiron unit that mimic the structure of the full H-cluster suffer from instability and low activity [8] . Full catalytic activity for proton reduction approaching the efficiency of the enzyme has only been achieved in hybrid constructs where the synthetic model (μ-(SCH 2 ) 2 NH)[Fe(CO) 2 (CN)] 2 2− has been inserted into the apo-[FeFe]-H 2 ase protein [9] , [10] . If the substantive goal of creating robust electrocatalysts in simple to assemble, earth-abundant materials is to be realized, we posit that a broader search for metal/ligand frameworks is needed. 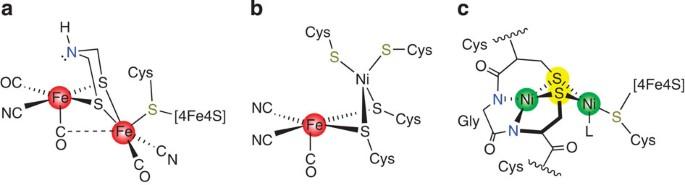Figure 1: Structures of bimetallic enzyme active sites. (a) [FeFe]-hydrogenase; (b) [NiFe]-hydrogenase; (c) Acetyl-CoA synthase. Figure 1: Structures of bimetallic enzyme active sites. ( a ) [FeFe]-hydrogenase; ( b ) [NiFe]-hydrogenase; ( c ) Acetyl-CoA synthase. Full size image The ubiquity of bimetallic active sites in biology provides a compelling reason to search for features that inform on the contributions of individual metals to the overall catalytic processes. The active site of [NiFe]-H 2 ase can be interpreted as a nickel dithiolate metalloligand bound to the Fe II (CN) 2 (CO) organoiron fragment through protein-bound cysteines, with a Ni–Fe distance of ca. 2.5–2.8 Å (ref. 11 ) ( Fig. 1 ). As a metallodithiolate ligand the (RS) 2 Ni(μ-SR) 2 donor is reminiscent of the cys-gly-cys, Ni II N 2 S 2 motif of acetyl-CoA synthase, a more obvious metallodithiolate ligand that binds a second nickel, however, at 3.0 Å, beyond metal–metal bonding distance [12] . ( Fig. 1 ) Of significance to our study below is an NiN 2 S 2 ·Fe(NO) 2 complex of Pohl et al. [13] that was reported as a mimic of the [NiFe]-H 2 ase site in 1997. Recognizing the need for redox flexibility in terms of delocalization in storage, speciation on demand by a proton and charge capacity, here we combine the metallodithiolate-as-ligand concept to a second iron within a setting of nitrosyl ligands, producing a novel diiron trinitrosyl complex, [(NO)Fe(N 2 S 2 )Fe(NO) 2 ] +/0 , and explore its properties in stable oxidized and reduced levels, 1 + and 1 red , respectively. When bound to a transition metal, nitric oxide is known to exhibit strong covalency especially as compared with CO/CN − /PR 3 ligands; this covalency has a significant impact on the functional oxidation state of the metal centre [14] . Thus, along with ν (NO) infrared data, the spectral signatures available from Mössbauer and EPR spectroscopies are appropriate probes of communication between nitrosylated metal sites. Molecular structures of 1 + and 1 red demonstrate the accommodation of redox level changes in such bimetallic complexes that involve both irons and the electronically versatile, or ‘non-innocent’, NO ligand [15] , [16] . Such regulation of electron density within a stable small molecule that responds to added electrons and protons offers a unique approach to bio-inspired diiron hydrogenase active site models, based on which potential electrocatalysts could be developed. Synthesis and characterization While exploring the NO release ability of an unusually stable trinitrosyl iron complex, using a [(bme-dach)Fe] 2 complex (bme-dach=N,N′-bis(2-mercaptoethyl)-1,4-diazacycloheptane) as an efficient NO-trapping agent, we isolated the stable, dark-brown complex cation 1 + , as its BF 4 − salt ( Fig. 2 ) [17] . The molecular structure ( Fig. 2b ) was interpreted as a combination of a (bme-dach)Fe(NO) unit, a known product of [(bme-dach)Fe] 2 dimer cleavage by free, gaseous NO ref. 18 ), that serves as a metallodithiolate donor ligand to an {Fe(NO) 2 } 9 unit (Enemark–Feltham notation [19] ). Such an electron count represents the oxidized form of a d i n itrosyl i ron c omplex (DNIC). While monomeric DNICs at the {Fe(NO) 2 } 9 redox level, such as those that are biologically relevant, have a prominent g =2.03 EPR feature [20] , complex 1 + is diamagnetic, apparently resulting from antiferromagnetically coupled {Fe(NO) 2 } 9 and {Fe(NO)} 7 fragments, each with S =½ at an Fe—Fe distance of 2.786(1) Å. Subsequently, a convenient, one-pot synthesis of this dissymmetric diiron complex ( Fig. 2a ) made use of the reaction of Fe(CO) 3 (NO) − as precursor to a (proposed) transient Fe(CO) 2 (NO) 2 + species that readily releases CO and NO, the latter accounting for the (bme-dach)Fe(NO) unit [21] . This in situ production of both parts of the bimetallic complex suggested thermodynamic stability for 1 + , a common requisite shared by many practical molecular electrocatalysts. 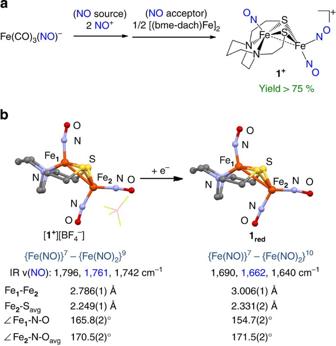Figure 2: Synthesis and characterization of complexes 1+and 1red. (a) Reaction scheme for the synthesis of1+. (b) Molecular structures of complex1+and1redas ball-and-stick renditions. (The BF4−counterion of1+is shown in wireframe view.) Thermal ellipsoid plots, structural packing diagram, crystal information and a full list of metric parameters of1redare provided asSupplementary Figs 1 and 2andSupplementary Tables 1 and 2. Figure 2: Synthesis and characterization of complexes 1 + and 1 red . ( a ) Reaction scheme for the synthesis of 1 + . ( b ) Molecular structures of complex 1 + and 1 red as ball-and-stick renditions. (The BF 4 − counterion of 1 + is shown in wireframe view.) Thermal ellipsoid plots, structural packing diagram, crystal information and a full list of metric parameters of 1 red are provided as Supplementary Figs 1 and 2 and Supplementary Tables 1 and 2 . Full size image The cyclic voltammogram of complex 1 + displays two redox events at E 1/2 =−0.78 and −1.41 V (versus Fc + /Fc) in CH 2 Cl 2 solution, shown in Supplementary Fig. 3a . The good linearity of the plot of current response to the square root of scan rates, 50–1,000 mV s −1 , indicates that the two events are fully reversible with electron transfer limited by diffusion control ( Supplementary Fig. 3b ) [22] , [23] , [24] . The cyclic voltammograms of ( i -Pr-NHC) 2 Fe(NO) 2 (ref. 25 ) ( i -Pr-NHC=1,3-diisopropylimidazol-2-ylidene) and (bme-dach)Fe(NO) [18] , taken as exemplars of the individual components of complex 1 + , are shown in Supplementary Fig. 3c,d . Both display a single reversible redox event within the range of complex 1 + . The former, isolated in reduced form, has a {Fe(NO) 2 } 9/10 couple centred at −0.77 V, while the latter mono-nitrosyl iron complex has an {Fe(NO)} 7/8 couple centred at −1.70 V. Hence, it is reasonable to assign the more positive couple of complex 1 + to the DNIC portion of the bimetallic complex, while the more negative is largely due to the Fe(NO) in N 2 S 2 ligation. As both the ( i -Pr-NHC) 2 Fe(NO) 2 and (bme-dach)Fe(NO) complexes have been identified in two redox levels, and as the redox events in compound 1 + are fully reversible, we endeavoured to isolate a reduced version of 1 + produced by bulk chemical means. As reductants, both cobaltocene (Cp 2 Co, E 1/2 =−1.33 V) [26] or Li + Et 3 BH − react with 1 + resulting in a colour change from red-brown to olive green with concomitant shifts by ca. 100 cm −1 of the three ν (NO) IR absorptions to lower values. From the ν (NO) intensity pattern of complexes 1 + and 1 red , as well as the band separation, the IR bands at 1,796 (m) and 1,742 (vs) cm −1 of 1 + and 1,690 (m) and 1,640 (s) cm −1 of 1 red are assigned to the Fe(NO) 2 unit, while the central ν (NO) band at 1,761 (s) cm −1 of 1 + and 1,662 (vs) cm −1 of 1 red derives from the Fe(NO) portion. 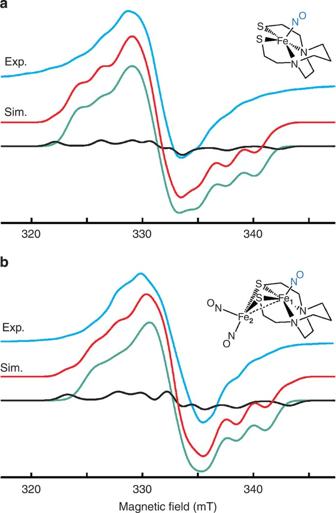Figure 3: X-band CW EPR spectra. (a) [(bme-dach)Fe(NO)] and (b)1redin CH2Cl2at 10 K. The blue line represents the experimental data, while the red line is the total simulation taking into account 90% of species I (green) and 10% of species II (black) (seeSupplementary Table 4). Measurement conditions: modulation amplitude=0.5 mT; power=0.04 mW; frequency=9.472 GHz for (a) and 9.474 GHz for (b). Computational results support this assignment of ν (NO) IR positions ( Supplementary Table 3 ). Dark-green crystals of complex 1 red of X-ray diffraction analysis quality were obtained from tetrahydrofuran (THF) layered with pentane at −35 °C (see Supplementary Data 1 ). Figure 2b shows the molecular structures of the two diiron complexes, 1 + (from the earlier study) [17] and 1 red . Note that the overall butterfly shapes of the diiron complexes are the same, consistent with the similar ν (NO) infrared absorption pattern and band separation, vide infra . The average Fe 1 -S distance within the N 2 S 2 -binding site is maintained at ca. 2.25 Å in 1 + and 1 red ; however, there is a slight ( ca. 0.1 Å) elongation of the average Fe 2 -S distance in the reduced form. In both complexes, the plane of the Fe(NO) 2 unit is perpendicular to the N 2 S 2 plane and eclipses the Fe 1 -NO vector; that is, the (NO)Fe 1 Fe 2 (NO) 2 atoms are coplanar. The Fe-Fe distance increases by ca. 0.22 Å from 1 + to 1 red , with contributing factors being the displacement of the Fe 1 (NO) unit out of the N 2 S 2 plane (0.524 Å in 1 + and 0.550 Å in 1 red ) and the decrease of the S-S distance (3.253 Å in 1 + and 3.132 Å in 1 red ), which opens up the ∠ Fe 1 -S-Fe 2 by ca. 6°. Other differences of note are the ∠ Fe 1 -N-O angle in 1 + of 165.8° that changes to 154.7° in 1 red . As the ∠ Fe-N-O of the free (bme-dach)Fe(NO) metallodithiolate ligand is 148(2)°, this metric suggests that the electron density drained from the Fe(NO) unit via the bridging thiolates in 1 red is less than that in 1 + ; that is, the nitrosyls act in concert to accommodate the redox level that is largely changing within the Fe(NO) 2 unit. Attempts to further reduce 1 red using stronger reductants such as KC 8 or Na + (benzophenone − ) resulted in decomposition and rearrangement with the only identifiable product being reduced Roussin’s red ester (see Supplementary Methods for details) [18] . The isolated mono-nitrosyl component of 1 + , (bme-dach)Fe(NO), is paramagnetic, as is 1 red , obtained by one-electron reduction of 1 + . The CW EPR spectrum of (bme-dach)Fe(NO) in CH 2 Cl 2 is remarkably similar to that of 1 red ( Fig. 3 ). Both spectra can be simulated by assuming an S =1/2 system with hyperfine coupling to a single nitrogen. 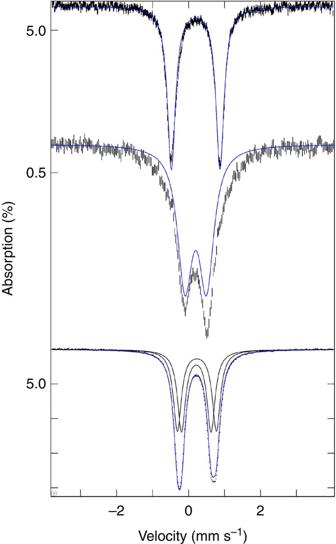Figure 4: Mössbauer spectra. Solid samples of (a) (bmedach)Fe(NO) at 150 K; (b) [(PhS)2Fe(NO)2]−at 6 K and (c) complex1+BF4−at 5 K, in 0.04 T applied field. The dotted and hash mark spectra are the data, solid (δ1=0.21 mm s−1) and dashed (δ2=0.23 mm s−1) lines are spectral fits. The simulation details are given in Supplementary Table 4 . The components of the g -tensor for 1 red are slightly smaller as compared with those of (bme-dach)Fe(NO). The presence of the second iron centre, Fe 2 , causes this perturbation, which apparently indicates that there is less σ donation to Fe 1 . Distortion of the Fe 1 -NO moiety from linearity would lead to changes in the strength of the interaction of the unpaired electron and nitrogen nucleus (NO) [27] . It should be noted that the spectrum of 1 red is best simulated with two species, one of which is a minor contributor ( ca. 10%). Both species are observed as well for (bme-dach)Fe(NO), whose X-ray crystal structure indicates two conformers of different Fe-N-O angles. This clearly shows that the electronic structures of (bme-dach)Fe(NO) as well as 1 red are similar, and the magnetic parameters of the Fe 1 core dominate the complete diiron compound 1 red . Thus, the first reduction of 1 + occurs on the Fe 2 moiety, and the spin is maintained on the Fe 1 core. Figure 3: X-band CW EPR spectra. ( a ) [(bme-dach)Fe(NO)] and ( b ) 1 red in CH 2 Cl 2 at 10 K. The blue line represents the experimental data, while the red line is the total simulation taking into account 90% of species I (green) and 10% of species II (black) (see Supplementary Table 4 ). Measurement conditions: modulation amplitude=0.5 mT; power=0.04 mW; frequency=9.472 GHz for ( a ) and 9.474 GHz for ( b ). Full size image The solid-state Mössbauer spectrum of cationic complex 1 + , in a 0.04 T applied field, presented in Fig. 4 can be well fitted with two quadrupole doublets, with equal areas, representing two individual iron sites. The Mössbauer data of the two mononuclear complexes that represent the components of {Fe(NO)} 7 -{Fe(NO) 2 } 9 1 + , the (bme-dach)Fe(NO), for the {Fe(NO)} 7 portion and the [PPN][(PhS) 2 Fe(NO) 2 ], for the {Fe(NO) 2 } 9 component, are shown for comparison ( Fig. 4 ). The differences between the parameters for the quadrupole doublets of 1 + and the matching mononuclear components are within the uncertainties of the fits for 1 + , given that such two-site fits are not unique. Nevertheless, the intrinsic iron features for each portion indeed represent together the complete diiron molecule, 1 + . (Note that we have used the bis carbene complex as reference for electrochemical studies described below since reduction of the [(NHC) 2 Fe(NO) 2 ] + yields a neutral species as does the 1 + to 1 red reduction process. In contrast, the [(PhS) 2 Fe(NO) 2 ] − species is assumed to be a better model for Mössbauer spectroscopy, where the electron-donating properties of the ligand donor atom predominate in the comparison.) It is worth noting that the parameters are surprisingly close to the range of those observed for the H ox state of [FeFe]-hydrogenase subcluster (0.1< δ <0.3 and 0.7<Δ E Q <1.2 mm s −1 ) [28] . Figure 4: Mössbauer spectra. Solid samples of ( a ) (bmedach)Fe(NO) at 150 K; ( b ) [(PhS) 2 Fe(NO) 2 ] − at 6 K and ( c ) complex 1 + BF 4 − at 5 K, in 0.04 T applied field. The dotted and hash mark spectra are the data, solid ( δ 1 =0.21 mm s −1 ) and dashed ( δ 2 =0.23 mm s −1 ) lines are spectral fits. Full size image Computational studies The structures, vibrational frequencies, energies and electrochemical features of complexes 1 + , 1 red and 1 − (second reduction of 1 + ) were calculated by a DFT methodology closely related to the one developed for metal nitrosyl complexes [29] (see Supplementary Note 1 for details). Good correlation with experimentally determined structural metrics and ν (NO) values for 1 + and 1 red supports the accuracy of this computational method ( Supplementary Table 3 ). Despite the reversibility of the couple in the cyclic voltammogram, the anion has not yet been isolated; 1 red is unstable to strong reducing agents. In order to define the 1 + / 1 red couple, the first reduction process in the cyclic voltammogram, the electronic and geometric structures of complexes 1 + and 1 red were calculated and the reduction potential of the former was determined. Previously, the coupling of {Fe 1 (NO)} 7 to {Fe 2 (NO) 2 } 9 in complex 1 + was described as a closed-shell singlet ground state [29] . Further investigation, however, finds a lower-lying, open-shell singlet. Therefore, the ground-state geometry of 1 + has been re-optimized as a mono-determinantal, broken-symmetry (BS) singlet that yields the Fe–Fe bond length in better agreement with the crystal structure (see Supplementary Table 3 ). The energy of this BS solution is lower than the closed-shell singlet and the triplet by 0.26 and 7.53 kcal mol −1 , respectively. The spin expectation value of the BS singlet of 1 + is 0.269 ( Table 1 ), an indication of significant diradical character with an electron on Fe 1 antiferromagnetically coupled to an electron on Fe 2 (see spin densities listed in Table 1 ). Table 1 Spin densities. Full size table Addition of one electron to complex 1 + leads to the experimentally observed doublet state of 1 red . With corrections for thermal motions and solvation (PCM, CH 2 Cl 2 ), the calculations predict a redox potential of −0.810 V from the BS 1 + to doublet 1 red (see Supplementary Methods ), which matches the experimental first redox event ( E 1/2 =−0.78 V). While 1 − has not been isolated, the calculation predicts a triplet ground state, with the singlet state being 9.18 kcal mol −1 higher in electronic energy. The calculated reduction potential for uptake of the second electron by 1 red is −2.08 V, which is ∼ 0.67 V more negative than the experimental value (−1.41 V; see Supplementary Tables 5–8 and Supplementary Note 1 ). Visualizations of the spin densities of 1 + , 1 red and 1 − are given in Fig. 5 . In all three cases, spin densities by Mulliken population analysis indicate that the unpaired spin densities are mainly localized on two irons and adjacent NO ligands with minor components on other atoms ( Fig. 5 and Table 1 ). The spin density changes during the reductions show that the first added electron is accommodated on the Fe 2 (NO) 2 moiety and the second added electron is accommodated on the Fe 1 (NO) moiety, which is consistent with electron accommodations assigned experimentally vide supra . 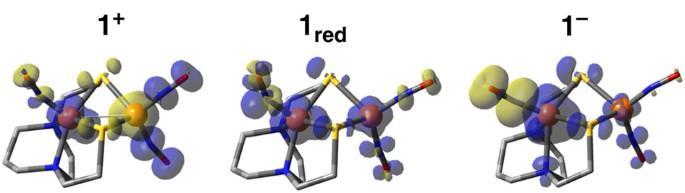Figure 5: Visualizations of the spin densities of complex 1+, 1redand 1−. The blue shading represents positive spin density (excess alpha spin) and the yellow shading represents negative spin density (excess beta spin). The colour of the shading changes on Fe2, when comparing1+and1red, because the excess beta spin density on Fe2is offset by adding an alpha electron during the first reduction. The second reduction enlarges the blue shaded area on Fe1, indicating the increase in alpha spin density. Figure 5: Visualizations of the spin densities of complex 1 + , 1 red and 1 − . The blue shading represents positive spin density (excess alpha spin) and the yellow shading represents negative spin density (excess beta spin). The colour of the shading changes on Fe 2 , when comparing 1 + and 1 red , because the excess beta spin density on Fe 2 is offset by adding an alpha electron during the first reduction. The second reduction enlarges the blue shaded area on Fe 1 , indicating the increase in alpha spin density. Full size image Consistent with the first added electron residing mainly on the Fe 2 (NO) 2 moiety, calculations show only slight changes in the bond distances between Fe 1 and its N 2 S 2 donors, in agreement with the experimental crystal structures. In contrast, the second added electron, predicted by theory to reside on the N 2 S 2 Fe 1 (NO) moiety, results in significant geometric alterations. The Fe 1 iron atom is further extruded from the plane formed by N 2 S 2 ; moreover, the distance between the N 2 S 2 mean plane and Fe 1 increases from 0.52 Å calculated for 1 red to 0.87 Å for 1 − , with Fe-S and Fe-N bond lengths elongated by ca. 0.27 and 0.12 Å, respectively. The elongated bond lengths indicate reduced donation from N 2 S 2 to Fe 1 in 1 − . In addition, significant changes in the ∠ Fe 1 (NO) angle are predicted by the calculation. In the first reduction, the calculated angle changes from 164.0° to 148.8° (as is observed experimentally) consistent with {Fe 1 (NO)} 7 within a metallodithiolate ligand that is less donating to the now reduced {Fe 2 (NO) 2 } 10 moiety. On addition of a second electron, computations predict a return to greater linearity of the mono-nitrosyl; ∠ Fe 1 (NO)=172.3°. Mulliken charge analysis shows the partial charge of the NO on Fe 1 (NO) changes by −0.012 and −0.564 in these two successive reduction events. That is, in the second reduction more electron density moves on the NO, yet it becomes more linear. Furthermore, there are unexpectedly large changes in the spin densities upon formation of 1 − ( Fig. 5 and Table 1 ) with alpha spin on Fe 1 of 2.142 (well above the expected value) and large beta spin density (−0.523) on its bound NO. All these lines of evidence indicate a more complicated change for the second reduction other than the simple addition of one electron to Fe 1 . Basically, the added electron and overall triplet spin produce a system that can be described as a high spin Fe 2+ ( d 6 ) antiferromagnetically coupled to a high spin NO − , which characteristically shows a linear Fe-N-O geometry (see Supplementary Fig. 4 ; Supplementary Table 9 and Supplementary Note 2 ) [30] . Proton reduction and electrocatalysis studies While complex 1 + does not react with HBF 4 in CH 2 Cl 2 solution, the isolated 1 red mixed with HBF 4 regenerates 1 + quantitatively as monitored by IR, with concurrent production of H 2 . Hydrogen was identified by dissolving the reaction headspace gas in CD 2 Cl 2 and recording its 1 H NMR spectrum, δ =4.59 (s) p.p.m. (ref. 31 ). ( Supplementary Fig. 5 ). Consistent with this observation, the first redox event ( E 1/2 =−0.78 V) in the cyclic voltammogram of 1 + shows a linear increase in current with added equivalents of HBF 4 ( Fig. 6a ). Bulk electrolysis further proves that the electrochemical response is at least partially attributed to the production of H 2 that was detected and quantified by gas chromatography (GC). Held at −1.05 V, the electrolysis provides a turn-over-number of 1.5 corresponding to a turn-over-frequency of 0.38 h −1 and a Faradaic efficiency of 36% in 4 h. The low efficiency is presumed to be due to catalyst decomposition during bulk electrolysis. 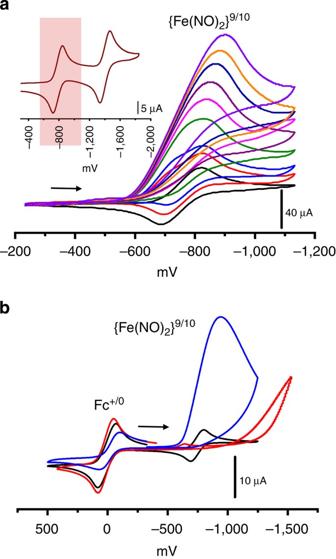Figure 6: Cyclic voltammogram diagrams. (a) First wave of1+with added HBF4(0–8 equiv) and the inset is the full CV of1+with the first wave highlighted. Note the change in slope at the addition of two equiv. of HBF4(blue), indicating the growth of a prewave or positive shift in the potential. (b) CV of cation1+(with no acid added, black); HBF4(without1+added, red); and cation1+with 50 equiv. of HBF4(blue). Conditions: scan rates of 200 mV s−1, complex1+in 2 mM CH2Cl2solution, under Ar, and referenced to Fc+/Fc. Arrows indicate direction of initiated scans. Figure 6: Cyclic voltammogram diagrams. ( a ) First wave of 1 + with added HBF 4 (0–8 equiv) and the inset is the full CV of 1 + with the first wave highlighted. Note the change in slope at the addition of two equiv. of HBF 4 (blue), indicating the growth of a prewave or positive shift in the potential. ( b ) CV of cation 1 + (with no acid added, black); HBF 4 (without 1 + added, red); and cation 1 + with 50 equiv. of HBF 4 (blue). Conditions: scan rates of 200 mV s −1 , complex 1 + in 2 mM CH 2 Cl 2 solution, under Ar, and referenced to Fc + /Fc. Arrows indicate direction of initiated scans. Full size image Note that the cyclic voltammograms in Fig. 6 have distinct features that will require a more thorough electrochemical study for their resolution, see the caption. We hypothesize that the slope change in the first reductive event of 1 + with added strong acid could be caused by the accumulation of the protonated counterpart of the catalyst—that is, 1·H + . With added equivalents of acetic acid (HOAc), the more negative redox event ( E 1/2 =−1.41 V) of complex 1 + shows a weak enhancement of current in its CV ( Supplementary Fig. 6 ) while the more positive wave is unperturbed. Given that at this potential and with weak acid H 2 was not detected by GC, the current response cannot be attributed to a completed catalytic cycle, vide infra . To probe the requirement of two irons for the electrocatalysis observed at −0.78 V, we have examined the current response of added acid to the individual components of this diiron complex that were described above. While the ( i -Pr-NHC) 2 Fe(NO) 2 complex shows a reversible wave at −0.77 V (ref. 25 ), addition of HBF 4 results in decomposition, with no electrocatalysis observed. The CV of unbound (bme-dach)Fe(NO) ( E 1/2 at −1.70 V) [18] is influenced by addition of HOAc, showing a slightly positive shift; however, there is no catalytic response ( Supplementary Fig. 3d,f ). Addition of HBF 4 to the mono-nitrosyl iron complex results in decomposition. Hence, the evidence strongly indicates that both irons are essential for the observed electrocatalytic behaviour of the 1 + / 1 red redox couple. The diiron cationic complex 1 + demonstrates the ability to accommodate one-electron reduction and crystallize in its neutral form of 1 red . From X-ray crystallography, subtle differences in geometry between 1 + and 1 red emphasize the interdependence of electronic and structural changes between the oxidized and reduced forms. The EPR spectrum of 1 red and supporting DFT computations provide a basis for a localized electron assignment as the antiferromagnetically coupled {Fe(NO)} 7 ·{Fe(NO) 2 } 9 unit of 1 + has changed to {Fe(NO)} 7 ·{Fe(NO) 2 } 10 in 1 red . While the added electron is on Fe 2 , components of both sides adjust to the additional negative charge. The reduced product 1 red is thermally stable but stoichiometrically reacts with strong acid to produce H 2 with return to 1 + , vide supra . While further detailed electrochemical/electrocatalytic studies are needed, the extant cyclic voltammograms and bulk electrolysis in this study suggest that when in contact with a supply of electrons and strong acid 1 red becomes active within an electrocatalytic, [CECE] cycle ( Fig. 7 ). While 1 red is inert to weak acid, its reduced partner, 1 − , assigned as {Fe(NO)} 8 ·{Fe(NO) 2 } 10 , and two electrons down from 1 + , has an electrochemical response in the presence of weak acid, however, with no H 2 detected ( Supplementary Fig. 6 ). 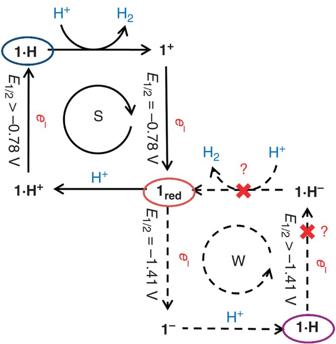Figure 7: Proposed catalytic cycles. The catalytic cycle (solid line and symbol ‘S’) in the strong acid is complete. The catalytic cycle in the weak acid (dashed line and symbol ‘W’) is incomplete, presumably due to incapability to transfer electron and/or proton to1·H. Figure 7: Proposed catalytic cycles. The catalytic cycle (solid line and symbol ‘S’) in the strong acid is complete. The catalytic cycle in the weak acid (dashed line and symbol ‘W’) is incomplete, presumably due to incapability to transfer electron and/or proton to 1·H . Full size image The interpretation of the electrochemical events with strong acid is consonant with proposals and mechanisms put forth for numerous detailed studies of the symmetrical (μ-SRS)[Fe(CO) 3 ] 2 complexes that have served as models of the [FeFe]-H 2 ase active site [2] , [4] , [32] , [33] , [34] . The advantage offered by complex 1 + is that its reduced partner, 1 red , has been fully characterized and is available as the entry into the catalytic cycle. A disadvantage of the 1 + /1 red system is that further reduction in order to increase basicity sufficient to utilize weak acids as protonating agents leads to immediate decomposition. Although a complete mechanism for sites of protonation and the production of H 2 will require considerably more experimental and computational work, some preliminary results are reported here. Upon the protonation of 1 red at Fe 2 , which calculations indicate is the best spot for protonation, the 1·H + is formed, to which addition of a second electron renders the production of H 2 with a strong acid. The synergism between these two sites is essential as neither of the complexes chosen as models of the separated species are electrocatalysts. With a weak acid, a second electron is needed before addition of the first proton. Predictive calculations suggest an increase in the basicity of 1 − compared with that of 1 red —that is, the acid dissociation constants of their conjugate acids differ by 13.5 p K a units, (see Supplementary Methods ) accounting for the interaction of 1 − with weak acids. It is noteworthy that the most basic site on 1 − is the nitrogen of Fe 1 (NO) instead of Fe 2 . Owing to the failure to detect any produced H 2 from the bulk electrolysis in the weak acid, the enhancement of electrochemical current in the CV ( Supplementary Fig. 6 ), which looks like a catalytic response at first glance, may actually have nothing to do with a completed catalytic cycle. The observed current enhancement is likely attributed to extra electron transfer to 1·H ; however, no further evidence is available to establish whether it is the failure of further electron or proton transfer to 1·H that terminates the proposed catalytic cycle ( Fig. 7 ). An alternative explanation to the current enhancement is offered in the caption of Supplementary Fig. 6 . Despite the limitations of this system, cation 1 + shows characteristics that are shared by good molecular electrocatalyst candidates: delocalization of electron density and a variety of protonation sites from which the ultimate trajectory of hydrogen atom coupling could be selected. This metallodithiolate/nitrosyl approach to biomimetics of the hydrogenase active site offers opportunity for modification of the carbon backbone of the N 2 S 2 ligand, as well as a choice of metals to be bound within the N 2 S 2 tight-binding site to be explored for optimization. Such opportunities for tuning electron uptake and distribution offer new vistas into which base metal electrocatalysis can be expanded. General experimental information All reactions and operations were carried out on a double-manifold Schlenk vacuum line under N 2 or Ar atmosphere. THF, pentane and diethyl ether were freshly purified by an MBraun Manual Solvent Purification System packed with Alcoa F200 activated alumina desiccant. The purified THF, CH 2 Cl 2 , pentane and diethyl ether were stored with molecular sieves under N 2 before experiments. The known complexes [PPN][Fe(CO) 3 (NO)] [35] and [(bme-dach)Fe] 2 (ref. 18 ) (bme-dach= N,N′ -Bis(2-mercaptoethyl)-1,4-diazacycloheptane) were synthesized by published procedures. The following materials were of reagent grade and were used as purchased from Sigma-Aldrich: cobaltacene, fluoroboric acid, nitrosonium tetrafluoroborate and lithium triethylborohydride. Physical measurements Infrared spectrometry was performed on a Bruker Tensor 27 FTIR spectrometer using 0.1-mm CaF 2 -sealed cells. X-band CW EPR measurements were carried out using an X-band Bruker ESP 300E spectrometer (with TE102 resonator) equipped with an Oxford Instruments helium flow cryostat (Oxford Instr., ESR910) and an ITC 503 temperature controller. X-band CW spectra were simulated using the EasySpin package [36] . Voltammograms were obtained using a standard three-electrode cell under an argon atmosphere at room temperature. Samples in CH 2 Cl 2 were run at a concentration of 2 mM with [n-Bu 4 N]PF 6 as the supporting electrolyte (100 mM) at a scan rate of 200 mV s −1 ; multiple scan rates are in Supplementary Fig. 3a . Bulk electrolysis experiments were performed at the Center for Molecular Electrocatalysis, Pacific Northwest National Laboratory and also at the Joint Center for Artificial Photosynthesis, California Institute of Technology. Details are provided below. Elemental analyses were performed by Atlantic Microlab Inc., Norcross, Georgia, USA. X-ray crystal structure analysis A Bausch and Lomb × 10 microscope was used to identify suitable crystals of the same habit. Each crystal was coated in paratone, affixed to a Nylon loop and placed under streaming nitrogen (110 K) in a SMART Apex CCD diffractometer (See Supplementary Data 1 ). The space group was determined on the basis of systematic absences and intensity statistics. The structures were solved by direct methods and refined by full-matrix least squares on F 2 . Anisotropic displacement parameters were determined for all nonhydrogen atoms. Placed at idealized positions, hydrogen atoms were refined with fixed isotropic displacement parameters. A list of programmes used is as follows: data collection and cell refinement, APEX2 (ref. 37 ); data reductions, SAINTPLUS Version 6.63 (ref. 38 ); absorption correction, SADABAS [39] ; structural solutions, SHELXS-97 (ref. 40 ); structural refinement, SHELXL-97 (ref. 41 ); graphics and publication materials, Mercury Version 2.3 (ref. 42 ). Synthesis of [(NO)Fe(N 2 S 2 )Fe(NO) 2 ][BF 4 ] (1 + ) The [PPN][Fe(CO) 3 (NO)] (0.28 g, 0.40 mmol), [NO][BF 4 ] (0.096 g, 0.80 mmol) and [(bme-dach)Fe] 2 (0.11 g, 0.20 mmol) reactants were loaded in a septum-sealed 50-ml Schlenk flask; 20 ml THF solvent were added by cannula. The reaction mixture was stirred for overnight at 22 °C; IR spectrum (THF solution): ν(NO) 1,796 (m), 1,761 (s), 1,742 (versus) cm −1 . The solution was filtered through Celite to remove insoluble solid and [PPN][BF 4 ]. Complex 1 + was isolated as a dark-brown solid after addition of pentane to the THF solution of 1 + [BF 4 ]. (Yield: 0.152 g, 75%.) Recrystallization in THF/pentane at −35 °C afforded crystals of complex 1 + [BF 4 ] suitable for X-ray crystallographic study, with results and properties being the same as those previously reported [17] . Elem. anal. found (calc’d for C 9 H 18 Fe 2 N 5 O 3 S 2 B 1 F 4 ) %: C, 21.33 (21.29); H, 3.58 (3.58), N, 13.82 (13.52). Synthesis of [(NO)Fe(N 2 S 2 )Fe(NO) 2 ] (1 red ) Under N 2 , LiHBEt 3 (0.40 ml of 0.1 M THF) was added dropwise to a THF solution of 1 (0.20 g, 0.40 mmol) at 0 °C in a septum-sealed 50-ml Schlenk flask. After stirring for 1 h, the IR monitor indicated no remaining starting material with new ν(NO) bands appearing at 1,690 (m), 1,662 (versus), 1,640 (s) cm −1 for 1 red (THF). The solution was filtered through Celite to remove precipitated LiBF 4 . Addition of pentane to the THF solution yielded a dark-green precipitate that was washed with pentane (3 × 20 ml) to further remove impurities (Yield: 0.090 g, 54%). Recrystallization in THF/pentane-diethyl ether at −35 °C afforded crystals of complex 1 red suitable for X-ray crystallographic study. Elem. anal., found (calc’d for C 9 H 18 Fe 2 N 5 O 3 S 2 ) %: C, 25.21 (25.73); H, 4.04 (4.32), N, 17.03 (16.67). Reaction of 1 red and HBF 4 Complex 1 red (0.42 g, 1.00 mmol) was loaded into a well-sealed vial and dissolved in THF (10 ml). A THF solution of HBF 4 .diethyl ether complex (0.162 g, 1.00 mmol) was syringed into the vial of 1 red . The reaction mixture was then stirred for 10 min. The headspace gas was slowly injected into a precooled CD 2 Cl 2 (0 °C) NMR tube. The IR spectral monitor revealed the formation of complex 1 + . The 1 H NMR measurement ( Supplementary Fig. 5 ) confirmed the formation of H 2 . Bulk electrolysis and analysis of produced H 2 Bulk electrolysis experiments were conducted in a three-necked 100-ml pear-type flask using a high-power BAS potentiostat (BASi power module PWR-3). One neck was closed by a rubber septum through which a copper wire was fed and connected to a cylinder of reticulated vitreous carbon that served as a working electrode for bulk electrolysis. The second and third necks were equipped with a reference electrode and a counter electrode was also fed through rubber septa. The reference electrode consisted of a AgCl-coated silver wire and 0.1 M n Bu 4 NPF 6 CH 2 Cl 2 electrolyte solution in a glass tube with Vycor frit. The counter electrode consisted of a Ni-Cr-coiled wire and a 0.1-M n Bu 4 NPF 6 /CH 2 Cl 2 electrolyte solution in a glass tube with glass frit. With these settings, the cell contains a 5-ml 0.1 M n Bu 4 NPF 6 CH 2 Cl 2 electrolyte solution of the compound, Fe 2 (NO) 3 (1 + as its BF 4 − , 5 mg, 2.0 mM), and a small amount of Cp 2 Fe ( ca. 1.8 mM) as internal reference under N 2 (1.0 atm). Before and after adding acid ( ca. 50 equivalents of Et 2 OŸHBF 4 , 50 ml, 1.0 M), two cyclic voltammograms were recorded to assure that the experiment was under catalytic conditions, and to determine the applied potential for bulk electrolysis. A second working electrode (1 mm PEEK-encased glassy carbon, Cypress Systems EE040) was employed to record cyclic voltammograms. Controlled-potential coulometry was performed at −1.05 V versus the Cp 2 Fe +/0 couple. After 8 C (corresponding to 4.1 calculated turnovers) of charge was applied over the course of 4 h, two 0.6-ml gas samples of the headspace in the flask were taken using two 1.0-ml gas tight syringes and then measured by an Agilent 6,850 gas chromatograph to quantify the percent of H 2 in the sample gas ( Supplementary Fig. 7 ). The Agilent 6,850 gas chromatograph was equipped with a thermal conductivity detector and was fitted with a 10 ft long Supelco 1/8′′ Carbosieve 100/120 column. The GC instrument was pre-calibrated to determine response factors for H 2 and N 2 using two H 2 /N 2 /CO/CO 2 mixtures of known composition. These measurements were obtained at the Pacific Northwest National Laboratory, Center for Molecular Electrocatalysis. A similar experiment with similar results was carried out at the Joint Center for Artificial Photosynthesis, California Institute of Technology. The latter found a significant deposit on the electrode surface for which an X-ray Photoelectron Spectrum of the surface post electrolysis detected the presence of Fe and S, confirmatory of the decomposition of catalyst during electrolysis. Computational methodology Metric parameters from the crystal structures of the complexes of 1 + and 1 red were imported into the AMPAC Graphical User Interface ( AGUI ) [43] and used as the initial geometries. Since no crystal structure is available for 1 − , the optimal geometry of doublet 1 red was used as the initial geometry for 1 − in optimization. All the optimal geometries were verified by frequency calculation to be a minimum by the absence of imaginary frequencies. The method applied is adopted from the recent methodology paper [29] with slight modifications. The specifications of calculations were set up by AGUI . The basis set applied is all-electron triple- ζ 6-311++G(d,p) [44] on all atoms. Both BP86 and TPSS functionals were reported to give similar results to those previously reported, so TPSS [45] was used. The calculations were made in Gaussian 09 (ref. 46 ). The lowest energy structure calculated for each species was set to 0 kcal mol −1 , and all other energies were scaled relative to this point. The Gibbs free energy of formation corrected by thermal motions and solvation model was used to calculate the standard electrode potential. The thermal correction at 298.15 K was calculated using the optimal geometry in gas phase by frequency calculation. Moreover, the solvation correction was calculated by comparing the electronic energies before and after the PCM solvation model of CH 2 Cl 2 (with specification keywords dis , rep and cav ) was applied on optimal geometry in the gas phase. The ferrocenium/ferrocene couple was used as a reference electrode in the calculation of standard electrode potential and the energy of this reference couple was calculated under the same condition. Contour plots for molecular orbital and spin density plots were generated in AGUI with an isosurface value of 0.04 a.u. (MO) or 0.005 a.u. (spin density), respectively. The Mulliken population analysis data were extracted from the output files of the calculations mentioned above. Accession codes: The X-ray crystallographic coordinates for structures reported in this Article have been deposited at the Cambridge Crystallographic Data Centre (CCDC), under deposition number CCDC940518 ( 1 red ). These data can be obtained free of charge from The Cambridge Crystallographic Data Centre via www.ccdc.cam.ac.uk/data_request/cif . How to cite this article: Hsieh, C.-H. et al. Redox active iron nitrosyl units in proton reduction electrocatalysis. Nat. Commun. 5:3684 doi: 10.1038/ncomms4684 (2014).